Sequencing of first-strand cDNA library reveals full-length transcriptomes Massively parallel strand-specific sequencing of RNA (ssRNA-seq) has emerged as a powerful tool for profiling complex transcriptomes. However, many current methods for ssRNA-seq suffer from the underrepresentation of both the 5′ and 3′ ends of RNAs, which can be attributed to second-strand cDNA synthesis. The 5′ and 3′ ends of RNA harbour crucial information for gene regulation; namely, transcription start sites (TSSs) and polyadenylation sites. Here we report a novel ssRNA-seq method that does not involve second-strand cDNA synthesis, as we Directly Ligate sequencing Adaptors to the First-strand cDNA (DLAF). This novel method with fewer enzymatic reactions results in a higher quality of the libraries than the conventional method. Sequencing of DLAF libraries followed by a novel analysis pipeline enables the profiling of both 5′ ends and polyadenylation sites at near-base resolution. Therefore, DLAF offers the first genomics tool to obtain the ‘full-length’ transcriptome with a single library. Massively parallel sequencing of RNA (RNA-seq) has revolutionized our understanding of transcriptomes [1] , [2] , [3] . Several library preparation methods for strand-specific sequencing of RNA (ssRNA-seq) have been developed in the recent past [3] , [4] , [5] , [6] , [7] , [8] . However, a majority of these methods involve the synthesis of second-strand cDNA after reverse transcription (RT) that can entail multiple artefacts, including the loss of information at the 5′ and 3′ ends of RNAs. In addition, the second-strand synthesis demands multiple subsequent steps, including sonication, end repair and dA-tailing for adaptor ligation [5] , [6] , [7] , [8] , which can lead to a loss of cDNA. A lack of information about TSSs and polyadenylation sites creates serious challenges in investigating the molecular mechanisms of gene regulation. Second-strand synthesis can initiate from either RNase-H fragments or the hairpin structure at the 3′ end of first-strand cDNA [9] , [10] , [11] . The sonication step for shearing double-stranded cDNA may lead to the trimming of both linear and hairpin-structured 5′ ends ( Fig. 1 ) and the 3′ ends carrying the poly(A) tail. The exonuclease activity of Escherichia coli DNA polymerase I also degrades the 3′ ends of the first-strand cDNA [11] . Second-strand synthesis from hairpin structures, subsequent sonication and end repair with T4 DNA polymerase may cause an artificial loss or gain of nucleotides (α-γ in Fig. 1 ) and create artificial chimeric cDNA species (β in Fig. 1 ). 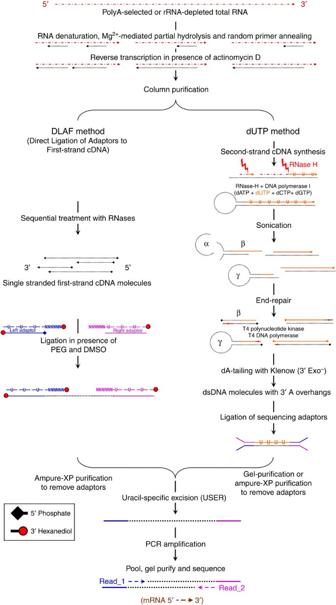Figure 1: A schematic comparison between the experimental workflows of the DLAF and dUTP methods. The rRNA-depleted or polyA-enriched RNA is reverse transcribed in the presence of actinomycin D. In DLAF, the double-stranded adaptors with overhangs are ligated to single-stranded cDNA molecules. The forward strands of adaptors containing dU residues are removed by USER, and the libraries are amplified by PCR. In the dUTP method, second-strand cDNA is synthesized in the presence of dUTP and fragmented by sonication, followed by the standard Illumina library preparation procedure and subsequent degradation of dU-containing second strands by USER. Read_1 indicates the reads in the direction of transcription. Read_2 indicates the reads sequenced from the other end of the cDNA molecules. Figure 1: A schematic comparison between the experimental workflows of the DLAF and dUTP methods. The rRNA-depleted or polyA-enriched RNA is reverse transcribed in the presence of actinomycin D. In DLAF, the double-stranded adaptors with overhangs are ligated to single-stranded cDNA molecules. The forward strands of adaptors containing dU residues are removed by USER, and the libraries are amplified by PCR. In the dUTP method, second-strand cDNA is synthesized in the presence of dUTP and fragmented by sonication, followed by the standard Illumina library preparation procedure and subsequent degradation of dU-containing second strands by USER. Read_1 indicates the reads in the direction of transcription. Read_2 indicates the reads sequenced from the other end of the cDNA molecules. Full size image Cap analysis of gene expression (CAGE) [12] , CAGE coupled with deep sequencing (DeepCAGE) [13] and sequencing of transcript leaders (TL-seq) [14] , which are based on the enrichment of RNA molecules with a 5′-cap structure, are currently the most reliable methods to identify transcription start sites (TSSs). However, CAGE tags and TL-seq predominantly represent the 5′-terminal base sequences of transcripts [12] , [14] ; therefore, most of the transcriptome is not represented in such libraries. In addition, the CAGE and TL-seq library preparation procedures are labour-intensive and require higher amounts of starting materials. NanoCAGE and CAGEscan, novel methods for enrichment of 5′-capped ends of RNA, have considerably reduced the amounts of RNA required for successful library preparation [15] , [16] . Likewise, a number of methods have been developed for the genome-wide profiling of polyadenylation sites [17] , [18] , [19] , [20] , [21] , [22] , [23] , [24] , [25] . These techniques provide important insights into tissue- and cell-type-specific usage of alternative polyadenylation sites. As most of these methods sequence only the poly(A) tail proximal 3′ region of mRNA, information from the non-polyadenylated RNA and the 5′ portion of polyadenylated RNA species is limited. Thus, to date, no ssRNA-seq method allows simultaneous profiling of 5′ and 3′ ends and expression of transcripts genome-wide, which hinders the deeper understanding of the complex transcriptome. Here we report a novel method for ssRNA-seq library preparation, in which we Directly Ligate Adaptors to the First-strand cDNA (referred to as the DLAF method). The omission of second-strand synthesis enabled a relatively shorter workflow and the preservation of information from both the 5′ and 3′ ends of the RNAs. A comprehensive comparison with the ‘dUTP method’, the current standard method for ssRNA-seq, revealed higher yield, complexity and mappability of DLAF libraries. In this study, we also compared DLAF with the ScriptSeq method [26] , [27] (Epicentre), which also does not involve second-strand cDNA synthesis. Compared with DLAF, ScriptSeq libraries showed a significant sequence bias and lower coverage of the RNA ends. Thus, DLAF represents a novel and versatile method for profiling and quantifying transcriptomes. Generation of the DLAF ssRNA-seq library In a recent systematic and comprehensive comparison of various methods for ssRNA-seq libraries, the dUTP method [8] outperformed other methods in multiple ways, including relative ease in experimentation and computational handling and a higher quality of data [28] . Since then, the dUTP method has become a standard in ssRNA-seq library preparation. The workflow of the dUTP method [8] is shown in Fig. 1 (right panel). The initial RT is primed by random oligonucleotides in the presence of actinomycin D to inhibit the DNA-dependent polymerase activity. Second-strand cDNA is synthesized in the presence of dUTP. The double-stranded cDNAs are then sheared by sonication, end repaired, dA-tailed and Y-shaped sequencing adaptors are ligated. The dUTP-containing second strand is degraded using uracil-specific excision reagent (USER) [29] enabling the determination of the genomic strand from which the transcripts were produced. In the DLAF method, first-strand cDNA synthesis is similar to that in the dUTP method, following which, the RNA is degraded by sequential treatment with ribonucleases (RNases) to yield single-stranded cDNA molecules ( Fig. 1 , left panel). A pair of double-stranded sequencing adaptors carries overhangs consisting of 5- or 6-random nucleotides ( Fig. 1 ). The overhang of each adaptor anneals to the end of a cDNA in a strand-specific manner, whereas the other strand of the adaptor ligates to the terminal nucleotide of the first-strand cDNA. The 3′ ends of the adaptor oligonucleotides are modified by hexanediol to limit concatenation. The ligation of the adaptors to the first-strand cDNA is carried out under an optimized condition, minimizing the GC content bias. The adaptor-ligated cDNAs are size-selected using solid phase reversible immobilization beads [30] , treated with USER to degrade the deoxyuridine-containing non-ligating strands of the adaptors, PCR-amplified and subjected to massively parallel sequencing. To avoid second-strand synthesis, the ligation of sequencing adaptors directly to the RNA molecules (RNA ligation) [3] , [31] or the use of a 3′-split adaptor [32] for RT can also be employed. We did not pursue these options because these techniques have a few limitations, including low library yields (see Supplementary Note 1 ). For a side-by-side comparison of the DLAF and dUTP methods, the first-strand cDNA samples were split equally for each method ( Fig. 1 ). The libraries were prepared using wild-type (WT) mouse embryonic stem (mES) cells and Kdm1a -deficient mES cells [33] in biological duplicates. For the dUTP libraries, we followed the published protocol ( Fig. 1 ) [8] , [28] , with minor modifications for an accurate comparison with DLAF (see Supplementary Note 2 ). Increased library yields The final yield of a library preparation method is an important indicator of its utility, especially when RNA is available only in small amounts. We first compared the relative yields of libraries prepared using the DLAF and dUTP methods with equal amounts of first-strand cDNA product. We quantified 2% of each library with quantitative and semi-quantitative PCR. On average, the DLAF method yielded approximately five times more library product (average ΔCt=2.53, P -value ( P )<0.01, two-tailed unpaired-samples Student’s t -test, Supplementary Fig. 1 ). The increased yield of the DLAF method is likely due to a decreased loss of cDNA in fewer steps and/or increased ligation efficiency using an optimized condition. Increased mappability and higher mapping to unique regions Multiplexed libraries were subjected to either single- or paired-end sequencing on an Illumina HiSeq 2000 instrument. We refer to the reads with the orientation of transcription as read_1 and the reads from the opposite orientation as read_2 throughout the present study ( Fig. 1 ). After standard demultiplexing and filtering, the reads were mapped to the mouse transcriptome and genome using TOPHAT [34] , allowing up to two mismatches. We first noted that the percentage of reads that mapped to the genome ( Table 1 , column: alignment rate, total) was higher for the DLAF libraries than the dUTP libraries. Higher mappability was consistent in WT (21.9% and 11.7% higher for read_1 and read_2, respectively) and Kdm1a -deficient mES cells (27.5 and 16.5% higher). Table 1 Mapping statistics of the DLAF and dUTP RNA-seq libraries. Full size table Next, we determined the percentage of reads that mapped to unique regions of the annotated genome ( Table 1 , column: alignment rate, unique). Interestingly, the percentages of such reads were substantially lower in Kdm1a -deficient mES cells than in libraries from WT mES cells, regardless of the methods used. The decrease in the percentages of the unique reads in Kdm1a -deficient mES cells could have been a result of an increased expression of murine endogenous retrovirus (MuERV-L) or other retrotransposable elements upon the loss of Kdm1a [33] . Importantly, the DLAF libraries showed a higher percentage of reads mapping to unique regions of the genome than did the dUTP libraries ( Table 1 , column: DLAF/dUTP, unique). A higher percentage of such reads in the DLAF libraries was common in WT and Kdm1a -deficient mES cells. One possible explanation for this difference is that the hairpin formation at the 5′ ends of the first-strand cDNA ( Fig. 1 ) [11] in the dUTP method might be more efficient for a repetitive sequence. Indeed, the DLAF/dUTP ratio of unique alignment was higher in the Kdm1a -deficient mES cells (approximately 55.3%) than in the WT mES cells (approximately 32.7%). Moreover, DLAF showed higher coverage of exonic regions, whereas reads from the dUTP libraries mapped more frequently to the intergenic regions ( Supplementary Fig. 2 ). Taken together, the DLAF libraries showed a consistently higher mappability to non-repetitive genic regions than did the dUTP libraries. Higher coverage at the 5′ ends of transcripts Next, we compared the coverage along the length of the genes. Using RNA-SeQC [28] , [35] , the genes were first categorized into top-, middle- and bottom-expressed groups based on their expression levels. Average coverage from the 5′ to the 3′ ends of the transcripts was then calculated for 5,000 middle-expressed genes for each percentile of their gene length. Strikingly, read_1 from the DLAF libraries showed a marked increase in the 5′-end coverage in contrast to an acute drop in coverage near the 5′ ends in the dUTP libraries ( Fig. 2 ). At the 3′ end, the dUTP and DLAF read_2 performed similarly. No significant difference was noted in the middle of the transcripts. The increasing coverage in the 3′→5′ direction could be attributed to RT in the same direction (see Supplementary Note 3 ).Thus, the DLAF libraries show a profound and specific improvement at the 5′ ends over the dUTP libraries. 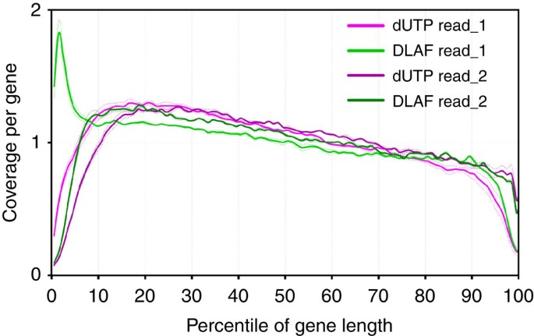Figure 2: RNA-SeQC analysis of coverage along the length of transcripts. Relative coverage for each percentile of gene length for the 5,000 middle-expressed genes in each library. Data are shown for individual replicates (dashed lines) and averaged replicates (solid line) from WT mES cells. RNA-SeQC coverage is shown normalized to the total number of reads mapping to the 5,000 middle-expressed genes. DLAF read_1 shows a distinct enrichment at the 5′ end of the genes, whereas dUTP read_1 shows depletion. Read_2 in both methods shows similar coverage throughout the length of the genes. Figure 2: RNA-SeQC analysis of coverage along the length of transcripts. Relative coverage for each percentile of gene length for the 5,000 middle-expressed genes in each library. Data are shown for individual replicates (dashed lines) and averaged replicates (solid line) from WT mES cells. RNA-SeQC coverage is shown normalized to the total number of reads mapping to the 5,000 middle-expressed genes. DLAF read_1 shows a distinct enrichment at the 5′ end of the genes, whereas dUTP read_1 shows depletion. Read_2 in both methods shows similar coverage throughout the length of the genes. Full size image Detection of TSSs with near single-nucleotide resolution To further characterize the increased coverage of 5′ ends, we plotted the first-sequenced nucleotide of read_1 (read-starts) along the annotated TSSs of the 5,000 middle-expressed genes in a strand-specific manner. Strikingly, a profound peak at exactly −1, 0 and +1 nucleotides relative to the annotated TSSs was observed for read_1 from the DLAF libraries ( Fig. 3a ), where we defined +1 nucleotide as the first base of a given transcript. In contrast, dUTP read_1 gave a minimal signal at the 5′ end. For DLAF read_1, a notable number of read-starts were also observed for up to 100 bases upstream of the TSSs. These upstream read-starts likely originate from either inaccurately annotated TSSs or tissue/cell type-specific TSSs. DLAF read_1 but not dUTP read_1 readily detected promoter antisense transcripts ( Fig. 3a ). Promoter antisense transcripts have been captured only after an enrichment of unstable RNA species [36] , [37] , [38] , [39] , [40] , [41] , [42] , [43] , such as nascent RNA or small RNAs. Taken together, DLAF enables sensitive detection of the TSSs of both mRNA and rare noncoding RNA species without any enrichment process. 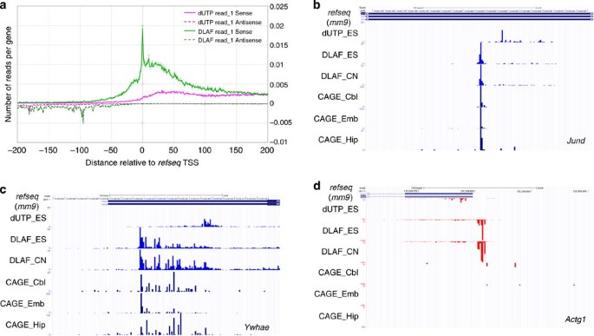Figure 3: DLAF results in an enrichment of TSSs at near-base resolution comparable to CAGE. (a) Coverage by the first-sequenced nucleotides of read_1 is plotted across the transcription start sites (TSSs) for the 5,000 middle-expressed genes from WT mES cells. Reads aligning to the antisense strand are plotted on the negativeyaxis. DLAF read_1 shows a profound enrichment at the annotated TSSs. (b–d) Comparison to DeepCAGE data. Starting positions of DLAF read_1 show the maxima at the 0 and -1 positions relative to the CAGE peaks. Peaks of DLAF read_1 near the TSSs ofJund(b) andYwhae(c) from mES cells (ES) and mouse cortical neurons (CN) coincide with the published CAGE peaks derived from the cerebellum (Cbl), embryo (Emb) and hippocampus (Hip)13. CAGE does not detect the TSSs of some genes, such asActg1(d). Coverage is normalized to the total non-rRNA and non-mtRNA reads for the dUTP and DLAF libraries. Figure 3: DLAF results in an enrichment of TSSs at near-base resolution comparable to CAGE. ( a ) Coverage by the first-sequenced nucleotides of read_1 is plotted across the transcription start sites (TSSs) for the 5,000 middle-expressed genes from WT mES cells. Reads aligning to the antisense strand are plotted on the negative y axis. DLAF read_1 shows a profound enrichment at the annotated TSSs. ( b – d ) Comparison to DeepCAGE data. Starting positions of DLAF read_1 show the maxima at the 0 and -1 positions relative to the CAGE peaks. Peaks of DLAF read_1 near the TSSs of Jund ( b ) and Ywhae ( c ) from mES cells (ES) and mouse cortical neurons (CN) coincide with the published CAGE peaks derived from the cerebellum (Cbl), embryo (Emb) and hippocampus (Hip) [13] . CAGE does not detect the TSSs of some genes, such as Actg1 ( d ). Coverage is normalized to the total non-rRNA and non-mtRNA reads for the dUTP and DLAF libraries. Full size image CAGE [12] and DeepCAGE [13] , the current standard techniques to profile TSSs, have provided invaluable insights into the mechanisms of gene regulation. For example, one CAGE study [12] revealed distinct groups of genes based on the modes of their promoter usages. Some genes use a single dominant nucleotide as a TSS (SP class), whereas another group is characterized as dispersed TSSs within 100 bases of DNA segments (BP class), suggesting their distinct regulatory mechanisms [12] . The peak of read-starts precisely at the annotated TSSs prompted us to compare DLAF data with the DeepCAGE data. We compared DeepCAGE tag clusters from mouse embryo, cerebellum and hippocampus [13] to the first-sequenced base of read_1, which were prepared from WT mES cells or mouse cortical neurons. As shown in Fig. 3b , the peak of read-starts in the DLAF library precisely matched to TSSs detected by CAGE for Jund and many other SP-class genes ( Supplementary Fig. 3 ). For a BP class gene, such as Ywhae ( Fig. 3c ), both the DLAF and CAGE libraries could detect a broad distribution of TSSs in the promoter region. The dUTP library largely failed to detect a TSS in any gene class. CAGE did not give signals for some highly expressed ubiquitous genes, such as Actg1 ( Fig. 3d ), Gapdh and Rpl18 ( Supplementary Fig. 3 ), whereas DLAF yielded discrete signals near their annotated TSSs. The absence of a CAGE signal for some highly expressed ubiquitous genes points to either an uncharacterized bias or a lower coverage in DeepCAGE. In addition to TSSs, DLAF also detects the 5′ ends of processed RNAs during biogenesis of microRNAs (miRNAs). MiRNAs are transcribed as long primary transcripts (pri-miRNAs) [44] , which are then processed by the RNase, Drosha, to generate one or more precursor-miRNAs (pre-miRNAs) [45] . These pre-miRNAs are then exported to the cytoplasm and processed into mature miRNAs [45] . As shown in Fig. 4a , DLAF but not dUTP libraries showed a prominent peak of read_1-starts that indicates a previously unknown TSS for the Mir290 pri-miRNA carrying multiple annotated miRNAs. Additional DLAF peaks coincided precisely with the 3′ ends of several miRNAs produced from the pri-miRNA and profiled by miRNA-seq ( Fig. 4 ). These peaks most likely represent the 5′ ends of the intervening RNA fragments between pre-miRNAs, generated by the cleavage of the pri-miRNA. Neither DLAF nor dUTP method detected the 5′ends of the mature miRNAs. We reason that mature miRNAs were lost during the size-selection step of the library preparation. It should be mentioned that DLAF can give a signal at the 0 (1 base upstream to TSS), −1 or −2 position relative to the 5′ end of RNA ( Supplementary Table 1 ) because of the non-templated nucleotide addition by Moloney murine leukemia virus reverse transcriptase or its variants [46] ( Supplementary Table 1 ). These results demonstrate that DLAF is a powerful method to profile the TSS and 5′ ends of transcripts generated by regulatory cleavages at near single-nucleotide resolution. 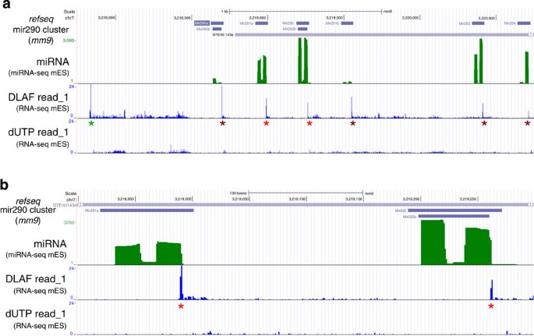Figure 4: DLAF detects non-capped 5′ ends of RNA generated by regulatory cleavage. (a) University of California, Santa Cruz (UCSC) genome browser view of the Mir290 cluster in WT mES cells showing the cleavage events of the primary miRNA (pri-miRNA) during miRNA biogenesis. Green: miRNA-Seq signal. Blue: first sequenced nucleotides of read_1 from the DLAF and dUTP libraries. A distal DLAF peak may represent a previously unknown TSS of pre-miRNA of the Mir290 cluster (green asterisk). Peaks of DLAF read_1-starts precisely match to internal cleavage sites on pri-miRNA (red and brown asterisks). Such peaks were not detected by the dUTP method. (b) Magnified view of two miRNAs, Mir291a and Mir292b (red asterisks). The peaks of DLAF read-starts are located at the nucleotide next to the 3′ end of each miRNA, indicating that DLAF results in the precise detection of 5′ ends of RNA fragments generated during processing of pri-miRNAs. Coverage is normalized to the total non-rRNA and non-mtRNA reads for the dUTP and DLAF libraries. Figure 4: DLAF detects non-capped 5′ ends of RNA generated by regulatory cleavage. ( a ) University of California, Santa Cruz (UCSC) genome browser view of the Mir290 cluster in WT mES cells showing the cleavage events of the primary miRNA (pri-miRNA) during miRNA biogenesis. Green: miRNA-Seq signal. Blue: first sequenced nucleotides of read_1 from the DLAF and dUTP libraries. A distal DLAF peak may represent a previously unknown TSS of pre-miRNA of the Mir290 cluster (green asterisk). Peaks of DLAF read_1-starts precisely match to internal cleavage sites on pri-miRNA (red and brown asterisks). Such peaks were not detected by the dUTP method. ( b ) Magnified view of two miRNAs, Mir291a and Mir292b (red asterisks). The peaks of DLAF read-starts are located at the nucleotide next to the 3′ end of each miRNA, indicating that DLAF results in the precise detection of 5′ ends of RNA fragments generated during processing of pri-miRNAs. Coverage is normalized to the total non-rRNA and non-mtRNA reads for the dUTP and DLAF libraries. Full size image 3′-End coverage and identification of polyadenylation sites To characterize the coverage at the 3′ ends of the genes, we plotted the read coverage of the DLAF and dUTP libraries near the annotated 3′ ends of the 5,000 middle-expressed genes in WT mES cells ( Fig. 5a ). Although DLAF read_1 showed a slightly higher coverage, DLAF read_2 exhibited a lower coverage than that of the dUTP libraries ( Fig. 5a ). 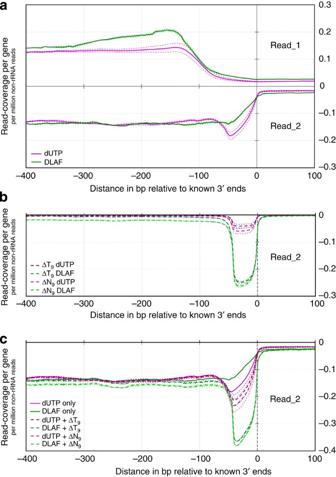Figure 5: Coverage of 3′ ends of genes and identification of polyadenylation sites via novel analysis. (a) Read coverage is shown near the annotated 3′ ends of the 5,000 middle-expressed genes in the DLAF and dUTP libraries. (b) Remapping reads after base trimming. Unmapped read_2 starting with a T9-stretch were selected; then, T9was removed (ΔT9) and remapped. As a control, data are also shown after trimming 9 bases (ΔN9) from all unmapped read_2. (c) Combined signals of initially mapped read_2 and remapped read_2 after base trimming. Coverage is shown as per gene per million non-rRNA reads. Data for individual replicates are shown as thin lines. Figure 5: Coverage of 3′ ends of genes and identification of polyadenylation sites via novel analysis. ( a ) Read coverage is shown near the annotated 3′ ends of the 5,000 middle-expressed genes in the DLAF and dUTP libraries. ( b ) Remapping reads after base trimming. Unmapped read_2 starting with a T 9 -stretch were selected; then, T 9 was removed (ΔT 9 ) and remapped. As a control, data are also shown after trimming 9 bases (ΔN 9 ) from all unmapped read_2. ( c ) Combined signals of initially mapped read_2 and remapped read_2 after base trimming. Coverage is shown as per gene per million non-rRNA reads. Data for individual replicates are shown as thin lines. Full size image During RT, we used an anchored oligo(dT) primer (T 9 VN, where V can be A, G or C), in addition to random primers, to retrieve the polyadenylated 3′ ends of the mRNA. We reasoned that the use of the oligo(dT) primer might have played a role in the lower coverage of DLAF read_2 near the 3′ end of the mRNAs. In a typical eukaryotic mRNA, the polyadenylation site represents the junction between a genome-encoded 3′ untranslated region (UTR) and a poly(A) tail; thus, reads originating from this chimeric sequence would not map to the genome. We postulated that computational trimming of poly(A) tails would enable these unmapped reads to align to the genome. To test this possibility, we first selected reads containing a 5′-T 9 sequence from unmapped read_2 in the initial alignment. Then, we trimmed T 9 and mapped them to the assembly again. Strikingly, the T 9 -trimmed reads (herein referred to ΔT 9 ) showed a profound signal only within 50 bases upstream of the annotated 3′ ends of the transcripts ( Fig. 5b ). As a control analysis, we also trimmed nine bases from all unmapped read_2, irrespective of the presence of a T 9 stretch (ΔN 9 ). For the DLAF libraries, ΔN 9 gave a comparable signal to ΔT 9 , suggesting that a significant fraction of unmapped read_2 in the initial alignment in the DLAF libraries was derived from polyadenylated 3′ ends of transcripts ( Fig. 5b ). Consistently, we found that a majority of the genomic regions represented by the DLAF or dUTP ΔT 9 reads showed the presence of known features of polyadenylation sites including the canonical polyadenylation sequences and the flanking U-rich sequences (see Supplementary Note 4 and Supplementary Fig. 4 ). As described earlier, after the initial alignment, dUTP read_2 showed slightly higher coverage of the 3′ ends than did DLAF read_2 ( Fig. 5a ). In contrast, the DLAF library showed dramatically higher coverage of the 3′ ends after the inclusion of the ΔT 9 or ΔN 9 reads ( Fig. 5c ). Interestingly, we observed cytosine as the most frequent base at the first nucleotide of ΔT 9 reads in DLAF but not dUTP libraries ( Supplementary Fig. 4b ). This cytosine likely represents −1 position at the cleavage sites, because the adenine of the canonical 5′-CA-3′ would anneal to the T 9 sequence and would be subsequently removed by the computational T 9 trimming. Consistently, the first base of ΔT 9 reads of the DLAF but not the dUTP libraries showed a profound peak at the -1 position of the annotated 3′ ends of mRNAs ( Supplementary Fig. 5 ). We speculate that either the 5′ to 3′ exonuclease activity of DNA polymerase I during the second-strand synthesis and/or the sonication step in the dUTP method might have partially or completely removed the poly(T) tails and part of the 3′ UTRs. This may also explain the higher coverage observed for dUTP read_2 in the initial alignment. The higher coverage in the DLAF libraries after the inclusion of the ΔT 9 or ΔN 9 reads suggests that the 3′ UTRs are largely intact in the DLAF libraries and, therefore, could be used to profile polyadenylation sites at near-base resolution with the novel analysis. End-to-end coverage of the transcriptome by DLAF Increased coverage at both ends of the mRNAs ( Figs 2 , 3 , 4 , 5 and Supplementary Fig. 6 ) suggests that DLAF could be a good tool to profile ‘full-length’ transcriptomes. To validate the full-length coverage quantitatively, we determined the number of genes covered by at least five reads within 50 bases of their annotated 5′ or 3′ ends using RNA-SeQC. For the 2,500 middle-expressed genes in the WT mES cells, DLAF read_1 showed a marked improvement in the coverage of the 5′ ends over the dUTP method (85.0% for DLAF versus 55.9% for dUTP, Fig. 6a ). For the 3′ ends, consistent with the averaged data in Fig. 5a , the initial mapping of dUTP read_2 covered a slightly higher number of genes (66.3%) than did DLAF (64.0%). However, when the mapped ΔT 9 or ΔN 9 reads were included, the DLAF libraries covered a higher number of genes than did the dUTP libraries (79.4% versus 69.4% with ΔT 9 and 78.5% versus 69.8% with ΔN 9 , Fig. 6a ). Similar trends were observed for both top- and bottom-expressed genes in the WT and Kdm1a -deficient mES cells ( Supplementary Figs 7 and 8 ). 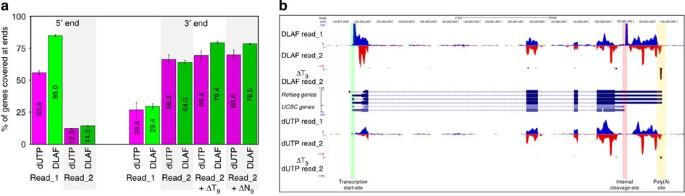Figure 6: DLAF results in end-to-end coverage of transcriptome. (a) Percentage of genes covered at 5′ and 3′ ends. RNA-SeQC data are shown for the 2,500 middle-expressed genes in WT mES cells. Data are shown for 12.5 million randomly selected non-rRNA and non-mtRNA reads. Average of two biological replicates is shown and error-bars indicate the range of data. (b) Image from the UCSC genome browser of theNanoglocus. DLAF read_1 shows a distinct coverage at the annotated TSS (green border) and an internal CS (pink border). Remapping of DLAF read_2 after ΔT9analysis identified the polyadenylation site (yellow border). Signals are normalized to the total number of non-rRNA and non-mtRNA reads from each library. Figure 6: DLAF results in end-to-end coverage of transcriptome. ( a ) Percentage of genes covered at 5′ and 3′ ends. RNA-SeQC data are shown for the 2,500 middle-expressed genes in WT mES cells. Data are shown for 12.5 million randomly selected non-rRNA and non-mtRNA reads. Average of two biological replicates is shown and error-bars indicate the range of data. ( b ) Image from the UCSC genome browser of the Nanog locus. DLAF read_1 shows a distinct coverage at the annotated TSS (green border) and an internal CS (pink border). Remapping of DLAF read_2 after ΔT 9 analysis identified the polyadenylation site (yellow border). Signals are normalized to the total number of non-rRNA and non-mtRNA reads from each library. Full size image The increased full-length coverage could be visualized in a genome browser at many individual loci ( Supplementary Fig. 9 ), including the Nanog locus ( Fig. 6b ) where DLAF read_1 but not dUTP read_1 showed coverage of the Nanog TSS. The DLAF ΔT 9 reads detected the poly(A) site of Refseq Nanog mRNA (NM_028016.3) with a single conspicuous peak, which was much weaker with the dUTP method ( Fig. 6b ). In addition, a profound peak in the DLAF read_1 but not the dUTP read_1 was noted precisely at the 3′ ends of previously annotated isoforms (NM_028016.2 and uc009dpo.1) of Nanog . It is plausible that Nanog mRNA undergoes previously uncharacterized cleavage to shorten the 3′ UTR, which was initially discovered in cancer cells [47] . Taken together, these data demonstrate that DLAF libraries define the precise positions of both 5′ and polyadenylated 3′ ends of transcripts genome-wide. High overall performance Reproducibility in expression profiling, evenness/continuity of coverage, strand specificity and library complexity are important criteria to assess the overall quality of an RNA-seq library [28] . In the previous comparative study, the dUTP method outperformed many other methods in terms of these criteria [28] . Using RNA-SeQC, we compared the overall performance of the DLAF and dUTP libraries prepared from either WT or Kdm1a -deficient mES cells across these criteria. As shown in Supplementary Fig. 10 , DLAF showed a high Pearson’s correlation to dUTP ( r >0.963 for WT and >0.949 for Kdm1a deficient mES cells), indicating that the gene expression profiles generated by the two methods were highly similar. Between the independent replicates, the DLAF and dUTP libraries showed equally high reproducibility, which was further confirmed by a lower coefficient of variation of gene expression, as calculated by Cuffdiff and CummeRbund [48] ( Supplementary Fig. 11 ). The DLAF libraries showed low average variations in evenness of coverage, which were slightly but significantly higher than those of the dUTP libraries (5.06% higher on average, P <0.01, two-tailed paired-samples Student’s t -test, Supplementary Fig. 12a ). The continuity of transcript coverage was defined as the fraction of transcripts’ length not covered by any reads; namely, gaps in coverage [28] . In both WT and Kdm1a -deficient mES cells, DLAF read_1 showed a lower gap percentage (21.77% on average, P <0.05, two-tailed paired-samples Student’s t -test) than did dUTP read_1, indicating a more continuous coverage. Read_2 from both methods performed similarly ( Supplementary Fig. 12b ). When we measured strand specificity, DLAF showed a higher strand specificity for read_2 of the WT mES cell samples ( Supplementary Fig. 13a ) and both read_1 and read_2 of the Kdm1a -deficient cells. The complexities of the libraries were calculated as fractions of reads with unique starting positions [28] . The DLAF libraries showed a significantly higher complexity in both read_1 and read_2 ( P <0.05, two-tailed paired-samples Student’s t -test, Supplementary Fig. 13b ). The sources of these improvements in strand-specificity and complexity are unclear. In summary, apart from a slightly lower evenness of coverage, the DLAF libraries exhibited higher overall quality across multiple performance metrics. Comparison of DLAF libraries with ScriptSeq v2 libraries Epicentre has developed a simple ssRNA-Seq method called ScriptSeq [26] , [27] , which does not involve second-strand cDNA synthesis. In ScriptSeq, the first-strand cDNA is generated using randomized oligonucleotides conjugated with Illumina’s reverse primer at the 5′ end. After RT, the 3′-ends of the single-stranded cDNA molecules are hybridized to a template-switching oligo, which consists of a ‘tagging sequence’, similar to the Illumina’s forward-primer sequence at the 5′ portion and randomized oligonucleotides at the 3′ portion. The 3′ end of the first-strand cDNA is then extended by a DNA polymerase to attach Illumina’s forward-primer sequence [26] , [27] . We sought to determine the similarities and differences between DLAF and ScriptSeq libraries. We prepared libraries using DLAF and a ScriptSeq v2 kit from E16.5 mouse embryonic cortex (mECx) in biological triplicates. To rule out differences arising from varied PCR conditions, we adopted the same PCR conditions as used for DLAF for the amplification of the ScriptSeq libraries. ScriptSeq libraries showed a significantly higher overall mapping rate and higher strand-specificity (see Supplementary Note 5 ). However, the ScriptSeq libraries showed lower library yields and a lower reproducibility. In addition, ScriptSeq libraries displayed significantly higher gap percentages and lower evenness of coverage, regardless of the expression levels, indicating a highly discontinuous coverage of transcripts (see Supplementary Note 5 for a possible explanation). These data demonstrate that, although the ScriptSeq had a higher mapping rate than did the DLAF, the mapped ScriptSeq reads represent lower reproducibility and a biased population of the transcripts. To test the hypothesis that the ScriptSeq method may create a sequence-bias, we extracted 50 bases of the genomic sequence immediately upstream of the read_1 and calculated their average base content. We found that these genomic fragments showed a distinct enrichment of the ‘GATCT’ sequence upstream of the ScriptSeq reads ( Fig. 7a ) but not the DLAF reads ( Supplementary Fig. 14 ). Strikingly, the tagging sequence of ScriptSeq template-switching oligo ends in GATCT at the junction with random oligonucleotides (Epicentre). Thus, lower library yield and more discontinuous and uneven coverage by the ScriptSeq libraries could be attributed to preferential hybridization of ScriptSeq oligonucleotides to RNA species that contain sequences complementary to the tagging sequence. 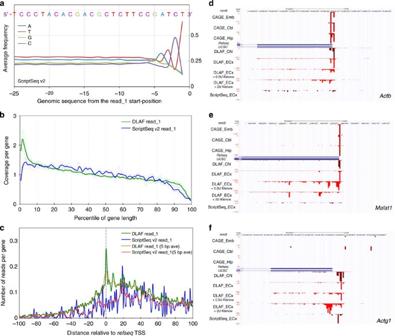Figure 7: Comparative analysis of ScriptSeq and DLAF libraries prepared from mouse embryonic cortices (ECx). (a) Base frequency in the genomic sequences upstream of read_1 in ScriptSeq libraries. Data are averaged from three biological replicates. The sequence shows a clear bias towards GATCT, which is similar to a part of template-switching oligo. (b) Coverage along the length of transcripts. RNA-SeQC coverage for each percentile of gene length is shown for the 5,000 middle-expressed genes. The coverage is normalized to the total number of reads mapping to the 5,000 middle-expressed genes in each library. (c) Distribution of the first-sequenced nucleotides of read_1. The first bases are plotted across the TSSs. Yellow (DLAF) and red (ScriptSeq) lines are 5-base moving average. DLAF read_1 but not ScriptSeq shows a peak around +1, 0 and −1 positions. Inbandc, dashed and solid lines denote individual and averaged replicates obtained from 5,000 middle-expressed genes. (d–f) Comparison to DeepCAGE data. Read_1-start positions of ScriptSeq and DLAF are shown forActb(d),Malat1(e) andActg1(f) loci. CAGE data are derived from the cerebellum (Cbl), embryo (Emb) and hippocampus (Hip)13. DLAF but not ScriptSeq peaks largely match with CAGE signals. DLAF libraries treated with Klenow show decreased and broader signals downstream of TSSs in a dose-dependent manner. Coverage is normalized to the total non-rRNA and non-mtRNA reads for the dUTP and DLAF libraries. Figure 7: Comparative analysis of ScriptSeq and DLAF libraries prepared from mouse embryonic cortices (ECx). ( a ) Base frequency in the genomic sequences upstream of read_1 in ScriptSeq libraries. Data are averaged from three biological replicates. The sequence shows a clear bias towards GATCT, which is similar to a part of template-switching oligo. ( b ) Coverage along the length of transcripts. RNA-SeQC coverage for each percentile of gene length is shown for the 5,000 middle-expressed genes. The coverage is normalized to the total number of reads mapping to the 5,000 middle-expressed genes in each library. ( c ) Distribution of the first-sequenced nucleotides of read_1. The first bases are plotted across the TSSs. Yellow (DLAF) and red (ScriptSeq) lines are 5-base moving average. DLAF read_1 but not ScriptSeq shows a peak around +1, 0 and −1 positions. In b and c , dashed and solid lines denote individual and averaged replicates obtained from 5,000 middle-expressed genes. ( d – f ) Comparison to DeepCAGE data. Read_1-start positions of ScriptSeq and DLAF are shown for Actb ( d ), Malat1 ( e ) and Actg1 ( f ) loci. CAGE data are derived from the cerebellum (Cbl), embryo (Emb) and hippocampus (Hip) [13] . DLAF but not ScriptSeq peaks largely match with CAGE signals. DLAF libraries treated with Klenow show decreased and broader signals downstream of TSSs in a dose-dependent manner. Coverage is normalized to the total non-rRNA and non-mtRNA reads for the dUTP and DLAF libraries. Full size image We then calculated the coverage across each percentile of their lengths. The ScriptSeq libraries showed lower coverage at both 5′ and 3′ ends than the DLAF libraries ( Fig. 7b and Supplementary Fig. 15 ). The lower coverage of the 3′ ends could be explained by the higher average insert size of the ScriptSeq libraries (ScriptSeq: ~375 bp versus DLAF: ~225 bp, data not shown), as read_1 would be farther from the 3′ ends of the transcripts and, therefore, less likely to be within 50 bases of the 3′ ends. In contrast to reproducible peaks of DLAF read_1-starts at the +1, 0 and −1 base positions relative to the annotated TSSs, the first bases of ScriptSeq read_1 showed the maximum average signal at ~20 bases downstream of the TSS, which slowly declined towards the TSS ( Fig. 7c ). Consistent with the earlier observation in mES cells, the peaks of read_1-starts of the DLAF libraries from mECx coincided precisely with the DeepCAGE peaks, whereas ScriptSeq libraries showed much lower signals at many loci, including Actb and Malat1 ( Figs 7d,e ). At other loci, such as Actg1 , the ScriptSeq read_1-starts showed a peak a few bases downstream from the TSS detected by DLAF or DeepCAGE ( Fig. 7f ). This loss of the terminal few bases at the 5′ ends in ScriptSeq libraries could be attributed to the sequence bias described earlier. We hypothesized that DLAF results in the enrichment of 5′ ends due to the preservation of the 3′ ends of cDNA, which could be degraded during second-strand cDNA synthesis by E. coli DNA polymerase I (ref. 11 ). To test this possibility directly, we examined the effect of the Klenow fragment (the 3′→5′ exonuclease component within DNA polymerase I (ref. 49 )) on the TSS detection in the DLAF libraries. We prepared DLAF libraries where RT reactions were treated with 0.5 or 2 U of Klenow fragment for 30 min at room temperature. Upon the Klenow treatment, the DLAF libraries showed lower signals at the TSSs and signals distributed further downstream of the TSSs in a Klenow dose-dependent manner ( Fig. 7d–f ). These results demonstrate that DLAF avoids the loss of cDNA ends that can be caused by E. coli DNA polymerase I carrying exonuclease activities during second-strand synthesis. In the ScriptSeq libraries, the coverage of 5′ ends by read_1 dropped at about the third percentile of gene length ( Fig. 7b ). This coverage pattern was noticeably improved compared with that of the dUTP libraries, which began declining at the tenth percentile ( Fig. 2 ). This improvement in the coverage of 5′ ends over the dUTP libraries is consistent with the idea that secondary-strand synthesis entails the loss of 5′ ends. RNA-sequencing libraries prepared using many of the current methods, including the dUTP method, show an underrepresentation of one or both transcript ends [28] . In this study, we developed a novel and relatively simple method, the DLAF, for preparing libraries for ssRNA-seq with markedly high coverage at both ends of transcripts. Our results indicate a versatile utility of DLAF for gene expression analysis and mechanistic study of gene regulation. DLAF libraries exhibit enrichment rather than restoration of lost information from RNA ends ( Figs 2 , 3 , 4 , 5 , 6 and Supplementary Fig. 6 ). Enrichment at the 5′ end of a transcript is likely because RT must end at the 5′ end of a transcript, where the reverse transcriptase falls off the RNA template. In contrast, in the middle of transcripts, RT can initiate or terminate at any position because RNA is randomly fragmented ( Supplementary Fig. 16 ). Likewise, an anchored oligo(dT) primer (T 9 VN) anneals specifically at the junction of the 3′ UTR and poly(A) tail; therefore, the polyadenylated 3′ end of the RNA is relatively enriched compared with other regions that are randomly primed ( Supplementary Fig. 16 ). The exact genomic position where the transcription of a gene starts is a critical piece of information in the study of mechanisms that control actions of RNA polymerases, such as recruitment, pausing and initiation. Genome-wide determination of TSSs has only been achieved using DeepCAGE [13] , TL-seq [14] , NanoCAGE and CAGEscan [15] methods. Utilizing smaller amounts of RNA and paired-end sequencing of longer fragments, CAGEscan appears to have resolved many of the limitations associated with previous CAGE analyses, as CAGEscan can assign newly discovered TSSs to downstream regions of the transcripts. The enrichment of 5′ end information in DLAF libraries complements these studies, as DLAF also enables the representation of 5′ distal portions of the transcripts in a library and, therefore, allows for simultaneous gene expression and additional transcriptome analyses, such as alternative splicing and polyadenylation. With the highly sensitive detection of 5′ ends of RNA, DLAF appears to be a useful technique to study alternative usage of TSSs in specific cell types ( Supplementary Fig. 17 ). However, in contrast to CAGE techniques and TL-seq, DLAF cannot differentiate a 5′-capped end of RNA from a 5′-end that lacks the cap structure; therefore, DLAF is limited in recognizing weak alternative TSSs that might be present downstream to a strong TSS. On the other hand, DLAF can be advantageous in profiling 5′ ends of RNA that lack the cap structure, such as prokaryotic mRNAs and RNAs that undergo regulatory cleavage [47] ( Figs 4 and 6b ). Meanwhile, the use of alternative polyadenylation sites is a prevalent mechanism of mRNA regulation in organisms from yeasts to mammals [50] . To map poly(A)-containing reads, several strategies have been employed, such as the use of a seed sequence or loosening the mapping stringency [24] , mapping reads to a transcripts database [18] and computationally removing the poly(T) tails [21] . These approaches rely on oligo(dT)-primed cDNA synthesis during RT; as a result, such libraries lack information from the 5′ portion of transcripts. In addition, these methods do not allow us to profile non-polyadenylated genes, such as mammalian histone genes, which can be readily detected in DLAF libraries ( Supplementary Fig. 18 ). Therefore, DLAF is the first genomics approach to simultaneously profile transcripts’ ends, including TSSs and alternative polyadenylation sites, with a single library. Single-cell RNA-seq has emerged as a landmark approach to understand the behaviour of individual cells instead of whole populations [51] , [52] , [53] , [54] . However, the current methods for single-cell RNA-seq cannot preserve the strand information. Improving yields, strand specificity and the quality of libraries will be an important step towards a genuine single-cell transcriptome. A high library yield and a relatively short experimental workflow of DLAF might be suitable for meeting the demands for analysing multiple single-cell libraries. However, further investigations are necessary to determine whether DLAF can be used to improve the transcriptome profiling of single cells. Cell culture Tissue culture dishes were coated with 0.1% gelatin (Sigma) for 30 min at 37 °C. The mES cells were cultured on the pre-coated dishes in high-glucose DMEM containing 15% ES-qualified fetal bovine serum (Chemicon), 2 mM glutamine, 1 × penicillin-streptomycin, 1 × non-essential amino acids, 10 mM HEPES, 143 μM β-mercaptoethanol (Sigma) and 1,000 U ml −1 of LIF (Chemicon) in a humidified incubator at 37 °C with 5% CO 2 . Cortices from E16.5 male mouse embryos were collected in HHGN dissection solution (Hanks’ balanced salt solution supplemented with 2.5 mM HEPES, 35 mM glucose, 4 mM sodium bicarbonate). Cortices were incubated with 0.1% trypsin in HHGN for 20 min at room temperature, quenched in Neurobasal media containing 10% fetal bovine serum and triturated under the presence of 0.01 mg ml −1 DNase I. Dissociated cells were suspended in Neurobasal media supplemented with 1 × B27 solution, 1 × penicillin-streptomycin, 0.5 mM glutamax and 25 μM β-mercaptoethanol. Cells from one cortex were plated on a 10-cm tissue culture dish pre-treated with 50 mg ml −1 poly- D -lysine hydrobromide (Sigma, MW=30,000–70,000). Cultures were maintained in a humidified incubator at 37 °C with 5% CO 2 . Half of culture media was replaced with new media every 5 days in vitro , and cells were harvested on 10 days in vitro . All reagents for cell culture were from Life Technologies unless mentioned otherwise. RNA isolation and removal of rRNA Total RNAs were isolated from approximately 10 million cells using TRIzol and 8 μg of each sample was subjected to rRNA depletion using RiboMinus Eukaryote Kit for RNA-seq (Life Technologies). RNA samples were treated with 6 U of Turbo-DNase (Life Technologies) in the presence of 80 U of Murine RNase Inhibitor from New England BioLabs (NEB) for 2 h at 37 °C. Although recommended otherwise by Life Technologies, rRNA depletion preceded DNase treatment to prevent any cation-mediated RNA hydrolysis during the DNase treatment. The DNase was removed using phenol-chloroform extraction, and RNA was precipitated and dissolved in 30 μl of water. RT for DLAF and dUTP libraries All oligonucleotides used in this study were procured from Integrated DNA Technologies (IDT). RT was carried out with random oligomers with a phosphate group at their 5′ end to obviate the phosphorylation step. The 30-μl RNA samples were mixed with 7 μl of the primer mix (25 μM 5′-NNNNNN-3′, 25 μM 5′-NNWNNWNN-3′ and 3 μM 5′-TTTTTTTTTVN-3′) and 7 μl of 10 × M-MuLV reverse-transcriptase reaction buffer (NEB). Partial RNA hydrolysis and annealing of random primers to RNA were achieved by heating the mixtures at 85 °C for 5 min and cooling them to 4 °C in a PCR thermal cycler at a standard ramp rate. RT was initiated by the addition of 26 μl of an ice-cold solution containing 4 μl of AffinityScript reverse transcriptase (Stratagene), 1 μl of Superase.In (Life Technologies), 3 μl of Murine RNase Inhibitor (NEB), 2 μl of 10 × T4 Polynucleotide Kinase buffer (NEB), 4.5 μl of 250 μM actinomycin D (Affymetrix) and 3 μl of 10 mM each of deoxynucleotides (dNTPs; NEB). The final RT conditions were 50 mM Tris (pH 8.3), 75 mM KCl, 6 mM Mg 2+ , 16 μM actinomycin D, 0.4 mM of each dNTPs, 2.5 μM 5′-NNNNNN-3′, 2.5 μM 5′-NNWNNWNN-3′ and 0.3 μM 5′-TTTTTTTTTVN-3′ (see Supplementary Note 6 for storage and usage of actinomycin D). The temperature of the reactions was increased slowly in a stepwise manner to avoid the dissociation of random primers from RNA molecules. The reactions were incubated at 2 °C for 2 min, 16 °C for 3 min, 0.1 °C s −1 to 25 °C, 25 °C for 10 min, 0.1 °C s −1 to 37 °C, 37 °C for 10 min, 0.1 °C s −1 to 42 °C, 42 °C for 45 min, 0.1 °C s −1 to 50 °C and 50 °C for 30 min. This was followed by cooling to 4 °C. The reactions were stopped by the addition of EDTA to a final concentration of 15 mM. They were then purified through a MinElute column (Qiagen) and divided equally for library preparation using either the dUTP or the DLAF method. DLAF library preparation To prepare the adaptors for ligation, six oligonucleotides with the sequences shown below were designed. Phos, U and C6 denote a 5′-phosphate modification, an internal deoxyuridine and a 3′-hexanediol modification, respectively. 1. LEFT_A: 5′-/5Phos/ AGATCGGAAGAGCGTCGTGTAGGG /C6/-3′ 2. LEFT_B5: 5′- CCCTACACGACGCUCTUCCGATCTNNNNN /C6/-3′ 3. LEFT_B6: 5′- CCCTACACGACGCUCTUCCGATCTNNNNNN /C6/-3′ 4. RIGHT_A: 5′- GGAGTTCAGACGTGTGCTCTTCCGATCCTG -3′ 5. RIGHT_B5: 5′- NNNNNCAGGAUCGGAAGAGCACACGUCTGAACTCC /C6/-3′ 6. RIGHT_B6: 5′- NNNNNNCAGGAUCGGAAGAGCACACGUCTGAACTCC /C6/-3′ The LEFT splint adaptor was prepared by annealing LEFT_A, LEFT_B5 and LEFT_B6 in a molar ratio of 1.95: 1:1. Similarly, the RIGHT splint adaptor was prepared by annealing RIGHT_A, RIGHT_B5 and RIGHT_B6. The LEFT and RIGHT splint adaptors ligate to the 3′ and 5′ ends of the first-strand cDNA, respectively ( Fig. 1 ). Purified first-strand cDNA was treated with 3 μl of RNase-H (NEB) for 2 h at 37 °C, followed by incubation with 2 μl of RNase-I f (NEB) for 2 h at 37 °C. The samples were column purified and treated with 1 μl of RNase-A (Fermentas) for 1 h at 37 °C and for an additional 1 h at 50 °C. The samples were then purified and eluted in 40 μl of IDTE buffer (10 mM Tris, 0.1 mM EDTA pH 8.0; IDT). The single-stranded cDNA samples were denatured for 3 min at 70 °C and quickly cooled on ice. The denatured cDNA samples were added to a 12-μl duplex mix containing 2.4 μl of 10 μM LEFT splint, 2.4 μl of 10 μM RIGHT splint and 1.2 μl of 10 × T4 DNA ligase buffer (NEB) at room temperature. The ligation was initiated by adding 50 μl of ligase mix containing 4 μl of 10 × T4 DNA ligase buffer (NEB), 1 μl of 10 μg/μl BSA (NEB), 2 μl of Quick T4 DNA ligase (NEB) and 33 μl of 2X Quick ligase buffer (NEB). After a 5-min incubation at room temperature, a PEG-DMSO mix containing 17.5 μl of 10 × T4 DNA ligase buffer, 17.5 μl of DMSO (NEB) and 35 μl of 50% PEG-8000 (NEB) was added. The mixtures were incubated for 2 h at 22 °C and then for 1 h at 30 °C. They were then column purified. The ligated samples were size-selected using 1.8 volumes of RNAClean XP beads (Beckman Coulter) with a 40-min incubation. The samples were incubated with 2 μl of USER (NEB) at 37 °C for 2 h to degrade the non-ligated strands of the splint adaptors and were then column purified. dUTP library In general, we followed the initial protocol for dUTP library preparation [8] , with minor modifications. For the second-strand cDNA synthesis, 40 μl of second-strand synthesis mix containing 6 μl of 10 × M-MuLV reverse transcriptase reaction buffer (NEB), 12 μl of 10 × phi29 DNA polymerase buffer (NEB), 18 μl of dNTP/dUTP mix (Fermentas), 3 μl of DNA polymerase I (NEB) and 1 μl of RNase-H (NEB) was added to 80 μl of purified first-strand cDNA samples, and mixtures were incubated at 16 °C for 2 h. E. coli DNA ligase was omitted during the second-strand synthesis (see Supplementary Note 2 ). Reactions were stopped by addition of EDTA to a final concentration of 20 mM, column purified and eluted with 60 μl buffer IDTE. Double-stranded cDNA samples were sonicated in a Bioruptor (Diagenode) for a total of 45 cycles of 30-s pulse with 30-s interval at high intensity at 4 °C. For end repair, we added 40 μl of reaction mix containing 10 μl of 10X NEBNext end repair reaction buffer (NEB) and 1 μl of NEBNext end repair enzyme mix (NEB). Samples were incubated at room temperature for 55 min followed by 5 min on ice and column purified into 60 μl of IDTE. Then, dA-tailing was initiated by adding 40 μl dA-tailing mix containing 10 μl of 10 × NEBNext dA-tailing Buffer (NEB) and 2 μl of Klenow Fragment (3′→5′ exo-) (NEB). Samples were incubated at 37 °C for 30 min and column purified into 40 μl of IDTE. An oligonucleotide dUTPLIG: 5′- GATCGGAAGAGCGTCGTGTAGGGAAAGAG U GACTGGAGTTCAGACGTGTGCTCTTCCGATC *T-3′ (where * represents a phosphorothioate bond) carrying a 5′ phosphate and an internal deoxyuridine (U) residue was synthesized, annealed and ligated to the dA-tailed double-stranded cDNA. The original oligonucleotide sequence [8] was modified to maintain the orientation of sequencing, similar to that of the DLAF libraries. To ligate the adaptors, we added 15 μl of 2 μM dUTPLIG adaptor and 84 μl of ligation mix containing 70 μl 2 × Quick Ligase Buffer, 12 μl IDTE and 2 μl Quick T4 DNA ligase to 40 μl dA-tailed libraries. After ligation for 1 h at room temperature, the cDNA libraries were column purified and size-selected using 1.6 volumes of RNAClean XP beads for 30 min, and the second strand was degraded by 2 h incubation with 2 μl of USER at 37 °C. Yield estimation and library amplification Two per cent of the library products were analysed by SYBR green-mediated quantitative PCR using QPCR_F1: 5′- CCCTACACGACGCTCTTCCGATCT -3′ and QPCR_R1: 5′- GGAGTTCAGACGTGTGCTCTTCC -3′. The same reactions were also amplified for 18 cycles in a conventional thermal cycler, and 10% were analysed using polyacrylamide gel electrophoresis. Based on the results, the libraries were amplified for 9 or 11 cycles of PCR for DLAF and dUTP, respectively, using MFWD: 5′- AATGATACGGCGACCACCGAGATCTACACTCTTTCCCTACACGACGCTCTTCC -3′ and reverse primer R x : 5′- CAAGCAGAAGACGGCATACGAGAT XXXXXX GTGACTGGAGTTCAGACGTGTGCTCTTCC -3′, where XXXXXX indicates the 6-nucleotide sequence for Illumina indexing oligonucleotide x for multiplexing. Next, 250–500 bp and 280–500 bp fragments were gel purified for the dUTP and DLAF libraries, respectively, for sequencing. Libraries preparation from mECx The cortices were dissected out from E16.5 male embryos and were dissolved in 800 μl of TRIzol. Handling of mouse complied with a protocol reviewed and approved by the University of Michigan’s University Committee on use and care of animals. After phase-separation, the supernatant was purified through Qiagen Mini Column. The rRNA was depleted from 4 μg of total RNA using RiboMinus Eukaryote Kit v2 (Life Technologies) with an average yield of approximately 320 ng RNA. The DNase I treatment and other purification steps were as described above. For the DLAF libraries, RT reactions were set up in a final volume of 25 μl containing 25 ng of rRNA-depleted RNA with the final reaction conditions as 50 mM Tris (pH 8.3), 75 mM KCl, 6 mM Mg 2+ , 10 μM actinomycin D, 0.4 mM of each dNTPs, 1 μM 5′-NNNNNN-3′, 1 μM 5′-NNWNNWNN-3′ and 0.12-μM 5′-TTTTTTTTTVN-3′. Treatment with RNases and other purification steps were as described above. The total reaction volume for each DLAF ligation was reduced to 100 μl with 5 pmol of each adaptor. ScriptSeq libraries from 25 ng of RNA were prepared using the ScriptSeq v2 kit (Epicentre) according to the manufacturer’s protocol. They were then column purified and size-selected using 1.8 volumes of RNAClean XP beads for 30 min. Two per cent of the library products were analysed by qPCR as described above. The same reactions were also amplified for 21 cycles in a conventional thermal cycler, and one-third volumes were analysed using polyacrylamide gel electrophoresis. Based on the results, the DLAF and ScriptSeq libraries were amplified as described above for 17 or 21 cycles of PCR, respectively. Next, 280–500 bp and 400–600 bp fragments were gel purified for the DLAF and ScriptSeq libraries, respectively, for sequencing. Sequencing, alignment and data analysis Libraries were sequenced for 50 bases (for mES cells and mouse cortical neurons) or 52 bases (for mECx) by an Illumina HiSeq 2000 instrument using standard oligonucleotides designed for multiplexed paired-end sequencing, except that DLAF read_2 was obtained using a specifically designed primer: 5′- GTGACTGGAGTTCAGACGTGTGCTCTTCCGATCCTG -3′. The mES libraries were subjected to both single-read and paired-end sequencing. Over the course of the analysis, we noticed that the third base from read_1 in the paired-end sequencing of the DLAF libraries had a reduced quality, likely because of a sequencer problem. Therefore, for the analysis of the DLAF library, we used read_1 data from the single-read sequencing and the read_2 from the paired-end sequencing (see Supplementary Table 2 ). Raw data were demultiplexed, filtered and converted to FASTQ files using standard procedure. Reads were mapped using TOPHAT v2.0.9 (ref. 34 ) to the mm9 genome and transcriptome, allowing for up to two mismatches. Coverage across percentiles of gene length, coverage of intragenic and intergenic regions, coverage of gene ends, evenness of coverage and continuity of coverage were calculated using RNA-SeQC [35] . The data were normalized with total non-ribosomal and non-mitochondrial RNA reads. The coefficient of variation of gene expression was calculated using Cuffdiff v2.1.1 and CummeRbund [48] . The complexity of the libraries was estimated as the fraction of 12.5-million randomly sampled, non-ribosomal and non-mitochondrial reads with unique starting positions using the rmdup utility of SAMtools [55] . The DeepCAGE data were lifted over from mm8 to mm9 using the UCSC liftOver utility. Read coverage and read-start coverage near TSSs and 3′ ends, the calculation of strand specificity and the comparison to CAGE were performed using our own scripts, which are available upon request. Preparation and analysis of miRNA-seq libraries Small RNA (<200 bases) was isolated from WT mES cells using the mirVana kit (Life Technologies) and the libraries were prepared using the Illumina’s small RNA Truseq kit according to the manufacturer’s protocol. Multiplexed libraries were sequenced from one end for 50 bases by an Illumina Hiseq 2000 instrument. After standard filtering, reads with the presence of Illumina’s reverse-PCR primer sequence were selected using the BBDuk utility of BBMap tools [56] and the adaptor sequence was removed from the reads. Only reads with shorter than 36 base inserts were mapped uniquely to mm9 assembly using bowtie v0.12.8 (ref. 57 ) allowing for up to one mismatch. How to cite this article: Agarwal, S. et al . Sequencing of first-strand cDNA library reveals full-length transcriptomes. Nat. Commun. 6:6002 doi: 10.1038/ncomms7002 (2015). Accession codes: Raw and processed sequence data files are available on the Gene Expression Omnibus (GEO) under accession GSE63424 . See Supplementary Table 2 for sample and sequencing run details.